Generation and control of polarization-entangled photons from GaAs island quantum dots by an electric field Semiconductor quantum dots are potential sources for generating polarization-entangled photons efficiently. The main prerequisite for such generation based on biexciton–exciton cascaded emission is to control the exciton fine-structure splitting. Among various techniques investigated for this purpose, an electric field is a promising means to facilitate the integration into optoelectronic devices. Here we demonstrate the generation of polarization-entangled photons from single GaAs quantum dots by an electric field. In contrast to previous studies, which were limited to In(Ga)As quantum dots, GaAs island quantum dots formed by a thickness fluctuation were used because they exhibit a larger oscillator strength and emit light with a shorter wavelength. A forward voltage was applied to a Schottky diode to control the fine-structure splitting. We observed a decrease and suppression in the fine-structure splitting of the studied single quantum dot with the field, which enabled us to generate polarization-entangled photons with a high fidelity of 0.72±0.05. The generation and the manipulation of on-demand entangled photons are crucial in the emerging fields of quantum cryptography [1] and quantum computation [2] . Hence, single semiconductor quantum dots (QDs) are considered potential sources of polarization-entangled photons through the radiative decay of biexcitons; a QD is initially excited to the biexciton state, and then it decays by a cascaded emission of two photons [3] . When the two exciton intermediate states are degenerate, the polarizations of the two photons are maximally entangled. However, they are not typically degenerated via the fine-structure splitting (FSS) owing to the asymmetries in the QD confining potential [4] , and its FSS energy (Δ FSS ) must be less than the radiative linewidth (Γ). It is also necessary that the cascade emission takes place with a high probability, which is expected to increase the visibility of the two-photon coincidence and the degree of entanglement [5] . Until now, the sources that use this scheme have been limited to In(Ga)As QDs [6] , [7] , [8] , [9] , [10] , [11] , [12] (with Γ of a few μeV) [13] , but the elongated shape and the strain in these QD systems induce a large in-plane anisotropy and a sizable Δ FSS (10–100 μeV) [14] . Because the typical Δ FSS observed for a QD exciton is usually larger than Γ, techniques to decrease Δ FSS must be used [13] , [15] , [16] , [17] . Here we take a different approach that satisfies these requirements by using the naturally bright [4] , [18] , [19] island QDs, made of a narrow GaAs quantum well (QW) with a monolayer thickness fluctuation [4] , [20] ; the FSS is suppressed by applying an electric field (E) in the forward direction onto a Schottky diode structure. In addition to the lack of strain, which affects Δ FSS , GaAs island QDs provide an oscillator strength that is one order of magnitude larger than that of self-assembled In(Ga)As QDs; hence, they present a higher emission probability [17] , [19] , [21] with a large Γ (23 μeV) [4] . This result arises because GaAs island QDs have a greater lateral extent area of the exciton than In(Ga)As QDs. Theoretically, GaAs island QDs are also expected to exhibit a smaller Δ FSS than In(Ga)As QDs because of the small electron–hole exchange energy, which is one order of magnitude smaller than that of self-assembled InAs QDs [22] . We observed a clear reduction of Δ FSS and a rotation of the exciton polarization axis caused by the electric field. At a certain value of the electric field, where Δ FSS is suppressed to below our detection limit, we obtained a high circular polarization degree of the exciton photoluminescence (PL) under a circularly polarized excitation. The polarization-dependent photon correlation measurements showed that applying electric fields to GaAs QDs makes it possible to manipulate the two-photon polarization state from the polarization-correlated state to the polarization-entangled state. GaAs island QDs in a Schottky device GaAs QDs were grown on an n-GaAs (100) substrate by molecular beam epitaxy. The QDs were created in the regions of one monolayer thicker than the other regions, which were formed during a 2-min growth interruption on both sides of the GaAs QW. 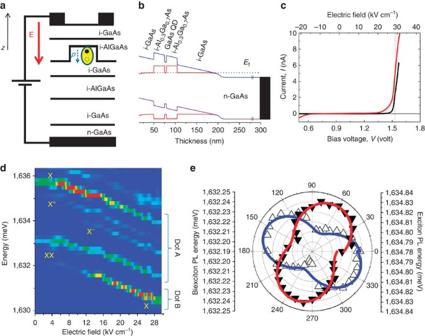Figure 1: Fabricated Schottky diode structure and QD photoluminescence characteristics on applying an electric field. (a) Schematics of the fabricated diode structure (not to scale). The thick red arrow denotes the direction of the applied vertical electric field E. The black arrow points to the sample growth directionz. The dotted arrow refers to the directional polarity of the QD exciton dipole momentp, and the yellow oval represents the hole component of the wavefunction below the electron in the dot. (b) One-dimensional simulation results of the device band alignment with the electric field (E=−45 kV cm−1) for the blue line and (E=0 kV cm−1) for the red line. (c)I−Vcharacteristics of the Schottky device in darkness (black line) and under 735 nm laser illumination (red line); the vertical dashed line refers to E=29.2 kV cm−1(whereI=5 nA). (d) Evolution of the photoluminescence spectra of two different GaAs quantum dots (dot A and dot B) with the electric field. For dot A, the recombination of the neutral exciton (X), the positively charged exciton (X+), the negatively charged exciton (X−) and the biexciton (XX) is shown. (e) Polar plot of the exciton (open-up triangles) and the biexciton (closed-down triangles) PL energies with the linear polarization angles, measured relative to, the sample's crystallographic axis, at E=18 kV cm−1. The solid blue (red) lines represent a fit to the exciton (biexciton) data, respectively, with a sinusoidal function, from which the fine-structure splitting magnitude and the exciton polarization direction were extracted. Figure 1a,b shows the fabricated Schottky diode structure and the simulation of the band diagram, respectively. No cavity structure was used to enhance the light-collection efficiency. An independent time-resolved μ-PL measurement was performed where the excitonic lifetime was found to be less than 300 ps, which reflects the fast radiative emission from our GaAs dots. We applied a forward bias voltage between the top gate metal contact and the bottom n-GaAs substrate (see Methods). The forward bias current ( I ) is quite small ( I <5 nA) owing to the presence of a thick Al 0.3 Ga 0.7 As barrier, which inhibits large currents from flowing through the device ( Fig. 1c ). Low temperature ( T =4 K) PL spectra are shown in Figure 1d as a function of E. The excitation and collection of PL was conducted through a 200-nm metal aperture, which was opened by electron beam lithography. For all measurements, we selected the excitation wavelength of 735–740 nm, which is about 40–50 meV higher than the exciton emission energy (approximately one longitudinal optical phonon energy of GaAs). Such an excitation wavelength is suitable to efficiently supply the photo-generated carriers to the QDs via phonon scattering. Figure 1: Fabricated Schottky diode structure and QD photoluminescence characteristics on applying an electric field. ( a ) Schematics of the fabricated diode structure (not to scale). The thick red arrow denotes the direction of the applied vertical electric field E. The black arrow points to the sample growth direction z . The dotted arrow refers to the directional polarity of the QD exciton dipole moment p , and the yellow oval represents the hole component of the wavefunction below the electron in the dot. ( b ) One-dimensional simulation results of the device band alignment with the electric field (E=−45 kV cm −1 ) for the blue line and (E=0 kV cm −1 ) for the red line. ( c ) I−V characteristics of the Schottky device in darkness (black line) and under 735 nm laser illumination (red line); the vertical dashed line refers to E=29.2 kV cm −1 (where I =5 nA). ( d ) Evolution of the photoluminescence spectra of two different GaAs quantum dots (dot A and dot B) with the electric field. For dot A, the recombination of the neutral exciton ( X ), the positively charged exciton ( X + ), the negatively charged exciton ( X − ) and the biexciton ( XX ) is shown. ( e ) Polar plot of the exciton (open-up triangles) and the biexciton (closed-down triangles) PL energies with the linear polarization angles, measured relative to , the sample's crystallographic axis, at E=18 kV cm −1 . The solid blue (red) lines represent a fit to the exciton (biexciton) data, respectively, with a sinusoidal function, from which the fine-structure splitting magnitude and the exciton polarization direction were extracted. Full size image Photoluminescence under applied electric fields The exciton PL emissions from two representative dots (dot A and dot B as indicated in Fig. 1d ) were observed with their redshift in the presence of the electric field. Here we focused on the result of dot A, where four emissions—an exciton ( X ), biexciton ( XX ), negatively charged exciton ( X − ) and positively charged exciton ( X + )—were detected. In addition to the linear and the superlinear responses of their PL intensities to the excitation power, the exciton and the biexciton emissions were assigned according to their opposite linear polarization ( Fig. 1e ). Thus, the exciton and the biexciton can be easily distinguished from X − and X + . The PL intensity dropped by 45% when E increased from 0 to 29.2 kV cm −1 , most probably owing to an increase of the field-assisted carrier tunnelling. Above E=29.2 kV cm −1 , the PL became significantly weak and broadened, which makes it difficult to determine Δ FSS at E>30 kV cm −1 (at these fields, I increases progressively above 10 nA ( Fig. 1c )). The observed dependence of the PL spectra on the electric field for other dots was similar to that represented in Figure 1d . Changes in polarization and FSS with the electric field The in-plane asymmetry of GaAs QDs is reflected in the polarization anisotropy exhibited by the integrated PL spectra of the exciton and the biexciton. By carefully following the evolution of the exciton and the biexciton PL energies with the polarization angle, we obtained a clear behaviour that could be fitted with a sinusoidal function, from which we extracted Δ FSS . The polarization axis of the PL was determined by the angle that represents the maximum splitting energy, and Δ FSS was measured with an accuracy of 2–3 μeV. 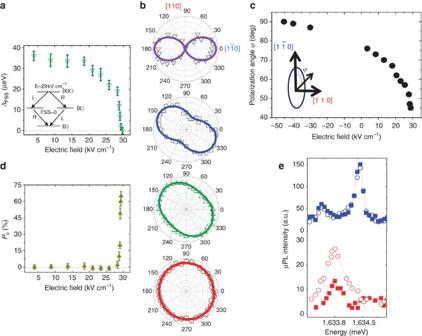Figure 2: Electric field-dependence of fine-structure splitting energy and QD exciton polarization. (a) Variation of ΔFSS(closed-down triangles) with the electric field. The inset shows a sketch of the biexciton–exciton cascaded emission for E~29 kV cm−1(ΔFSS~0). (b) Linear polarization dependence of the excitonXat various electric fields (from top): E=−45, 22, 27 and 29.2 kV cm−1, relative to, the sample's crystallographic axis. All polar plots have an axis scale increment of 10 μeV. The solid lines represent a fit to the data with a sinusoidal function. (c) Variation of the exciton polarization angleϕwith the electric field. The inset describes the angle ϕ relative to the crystal axis. The exciton PL emission cannot be seen when −30<E<−0.2 kV cm−1. (d) Evolution of the degree of exciton PL circular polarizationPc(closed-up triangles) with the electric field. (e) Circular polarization resolved detectionσ+(open-circles) andσ−(closed-squares) of the exciton PL spectra at two different electric fields: 23 kV cm−1(top) and 29.2 kV cm−1(bottom). Figure 2a shows a clear nonlinear change of Δ FSS with the electric field, where Δ FSS decreased from 38 μeV at E=0 to below our detection limit when the field approached 30 kV cm −1 . We studied five quantum dots; three of them showed a similar FSS suppression behaviour with the increase in the electric field. Moreover, on tuning Δ FSS over the measured range of the electric field, we observed a clear rotation of the exciton polarization axis. Figure 2b summarizes the relationship between the electric field and ϕ , which describes the orientation of the exciton polarization axis relative to the crystal axis . We found that as the field increased, the exciton polarization axis continuously rotated from ϕ =90°, where it aligned with the crystal axis [110] at E=−45 kV cm −1 , until it approached 45°, and it became independent of the polarization axis at E=29.2 kV cm −1 , where Δ FSS was minimized within our detection limit ( Fig. 2c ). Similar results have recently been reported for InAs/GaAs QDs using a large electric field of up to a few hundred kV cm −1 (ref. 12 ). Figure 2: Electric field-dependence of fine-structure splitting energy and QD exciton polarization. ( a ) Variation of Δ FSS (closed-down triangles) with the electric field. The inset shows a sketch of the biexciton–exciton cascaded emission for E~29 kV cm −1 (Δ FSS ~0). ( b ) Linear polarization dependence of the exciton X at various electric fields (from top): E=−45, 22, 27 and 29.2 kV cm −1 , relative to , the sample's crystallographic axis. All polar plots have an axis scale increment of 10 μeV. The solid lines represent a fit to the data with a sinusoidal function. ( c ) Variation of the exciton polarization angle ϕ with the electric field. The inset describes the angle ϕ relative to the crystal axis . The exciton PL emission cannot be seen when −30<E<−0.2 kV cm −1 . ( d ) Evolution of the degree of exciton PL circular polarization P c (closed-up triangles) with the electric field. ( e ) Circular polarization resolved detection σ + (open-circles) and σ − (closed-squares) of the exciton PL spectra at two different electric fields: 23 kV cm −1 (top) and 29.2 kV cm −1 (bottom). Full size image To confirm that Δ FSS approaches zero with the increase in the electric field, the QD exciton was excited by circularly polarized light with an energy of 40 meV above the exciton PL transition energy, and the exciton spin polarization was monitored by its PL circular polarization. Such one-longitudinal optical-phonon-assisted circularly polarized excitation induces a coherent superposition of both fine structure components of the exciton, which are split by Δ FSS . Analogous to the well-known Hanle effect, the degree of the exciton PL circular polarization ( P c ) is expected to increase when Δ FSS approaches zero [23] . Figure 2d shows the evolution of P c with the electric field. The polarized spectra of the exciton were plotted in Figure 2e for two different electric field strengths (E=23 and 29.2 kV cm −1 ). When the field strength increased, a strong increase in P c (65%) was observed, indicating that Δ FSS was greatly reduced at E=29.2 kV cm −1 compared with that at E=23 kV cm −1 . Quantum-confined Stark spectroscopy Now, we discuss the influence of the electric field on Δ FSS based on the QD exciton and biexciton Stark shift. A quantum confined Stark effect can introduce changes in the QD Coulomb interactions by modifying the overlap of the carriers' wavefunctions. Experimentally, we found that the emissions exhibited a quadratic shift according to the equation where E PL is the PL energy, and p and β are the permanent dipole and the polarizability of the state, respectively [24] . 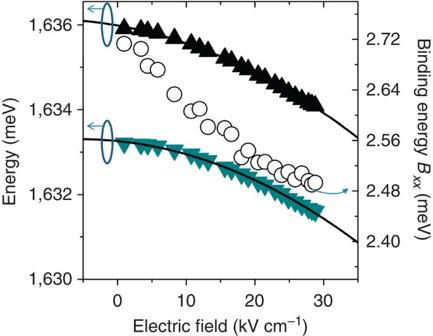Figure 3: Results of Stark spectroscopy measurements. PL peak positions of the exciton (closed-up triangles) and the biexciton (closed-down triangles) with the electric field. The electric field dependence of the biexciton binding energy (BXX), which is defined as the energy difference between the exciton and the biexciton emissions, is also shown and indicated by open circles. The left scale corresponds to the exciton and the biexciton data, and the right scale corresponds to theBXXdata; both scales are referred to by arrows. The solid lines represent the parabolic fits to the data, from whichpandβare extracted. The solid lines in Figure 3 show the results of the parabolic fit to the exciton and biexciton emission energies, from which we extracted p / e =−0.28±0.02 nm and β =−1.32±0.008 μeV/(kVcm −1 ) [2] for the exciton. A negative value of p indicates a permanent dipole moment along the −z direction; the hole wavefunction is located below the electron wavefunction ( Fig. 1a ). Figure 3: Results of Stark spectroscopy measurements. PL peak positions of the exciton (closed-up triangles) and the biexciton (closed-down triangles) with the electric field. The electric field dependence of the biexciton binding energy ( B XX ), which is defined as the energy difference between the exciton and the biexciton emissions, is also shown and indicated by open circles. The left scale corresponds to the exciton and the biexciton data, and the right scale corresponds to the B XX data; both scales are referred to by arrows. The solid lines represent the parabolic fits to the data, from which p and β are extracted. Full size image In Figure 3 , we plotted the electric-field dependence of the biexciton binding energy B XX , which is defined as the energy difference between the exciton and the biexciton emissions. A systematic reduction in B XX was observed. In a simple model, B XX can be expressed as: B XX =(−2 J eh + J ee + J hh ), where J eh is the electron–hole Coulomb interaction, and J ee and J hh are the electron–electron and the hole–hole Coulomb interactions, respectively. At E=0, a small spatial separation between the electron and the hole wavefunctions exists, giving rise to a permanent dipole moment. Because positive E and p are in the same direction as depicted in Figure 1a , the wavefunction separation increased with an increasing electric field, which led to a reduction in B XX by decreasing J eh . A decrease in B XX with the reduction of Δ FSS was previously reported for annealed InAs self-assembled QDs [25] . Although further study is required to understand the B XX reduction with the field, our results suggest that a positive electric field manipulates the electron–hole separation along the growth direction, and simultaneously modifies their lateral confinement; thus, the electric field enables the exciton dipole to rotate in the sample plane. Modulation of the exciton wavefunction by the electric field results in a decrease in the QD electron–hole overlap and a nonlinear change in the long-range component of the electron–hole exchange interaction, which strongly influences the FSS [26] . Although the electron–hole separation is expected at negative fields, we observed a sizable value of Δ FSS (=60 μeV) at E<−30 kV cm −1 ( Fig. 2b ), indicating the absence of a significant lateral modification of the exciton wavefunction at such field strengths. This observation is consistent with the lack of in-plane rotation of the exciton dipole within this electric field range ( Fig. 2b,c ). The polarity dependence may be related to the asymmetric nature of the two confining interfaces in our GaAs island QD [27] . It should be noted that the electric field dependence of Δ FSS in this case is qualitatively different from that of InAs/GaAs QDs, in which Δ FSS decreases linearly with the application of large reverse electric fields [12] . This difference might result from the 'weak' [4] , [28] lateral confining potential of our GaAs island QDs compared with the 'strong' lateral confinement of InAs/GaAs QDs (as a result, the carriers' wavefunctions in GaAs island QDs will be more sensitive to the applied electric fields than those of InAs/GaAs QDs). Polarization-resolved photon correlation measurements The suppression of the FSS by the electric field enabled us to examine the generation of polarization-entangled photons from the same dot. This generation relies on the biexciton–exciton cascaded emission, which can proceed along two paths as shown in the inset of Figure 2a : with a left-circularly-polarized (L) biexciton photon followed by a right-circularly-polarized (R) exciton photon, or vice versa. As Δ FSS approaches 0, it is impossible to distinguish which path the system has been followed, and the two photons should be emitted in the Bell state: Alternatively, the Bell state can be rewritten [1] , [9] in the linear polarization basis as or in the diagonal polarization basis as The first clear signature of the polarization-entangled photons from our GaAs island dot was observed in polarization-resolved photon correlation measurements ( Fig. 4a ). A clear photon bunching occurred for the collinearly polarized exciton and the biexciton photons emitted in the same cascade at zero delay time in the linear (VV) and the diagonal bases (DD), whereas in the circular basis, the bunching was observed only for the counter-circularly polarized (RL) photons. This result is expected for entangled photon pairs in the Bell state because the two-photon wavefunctions can be expressed as a superposition of the collinearly, co-diagonally or cross-circularly-polarized photon pairs [3] . The degree of entanglement was quantified using the degree of correlation (see Methods) ( Fig. 4b ), where the entanglement fidelity f + of the emitted photons projected onto the maximally entangled state was determined directly by combining the correlations measured in the linear, the diagonal and the circular polarization bases [29] . We found that the peak at the zero time delay yields a fidelity f + =0.72±0.05 ( Fig. 4c ) without any background light subtraction, which exceeds the threshold of 0.5 for a source emitting classically polarization-correlated states. Thus, the result proves that entangled photons were generated. 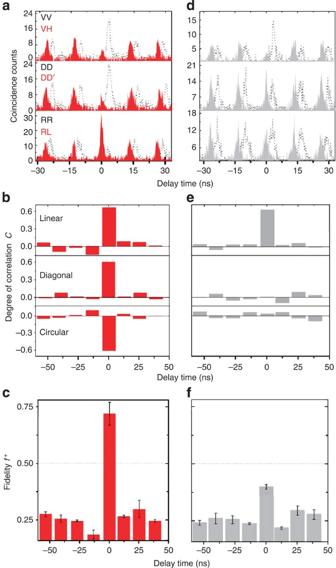Figure 4: Second-order cross-photon correlation histograms of biexciton–exciton photons. (a) Exciton and biexciton coincident counts for E=29.2 kV cm−1(ΔFSS~0) as a function of the delay time. The black dotted lines represent the coincident counts measured for photons of the same polarization, and the solid red lines show the orthogonal polarizations. (b) Degree of correlationCat E=29.2 kV cm−1for the linear (top), the diagonal (middle) and the circular (bottom) bases. (c) Fidelityf+for several central pulse periods at E=29.2 kV cm−1. (d) Exciton and biexciton coincident counts for E=18 kV cm−1(ΔFSS=30 μeV) as a function of the delay time. The black dotted lines represent the coincident counts measured for photons of the same polarization, and the solid grey lines show the orthogonal polarizations. (e) Degree of correlationCat E=18 kV cm−1for the linear (top), the diagonal (middle) and the circular (bottom) bases. (f) Fidelityf+for several central pulse periods at E=18 kV cm−1. The QD was excited quasi-resonantly by the 740 nm laser energy to minimize the recapture of the carriers into the dot. The black dotted histograms inaanddare time-shifted for clarity. The top, the middle and the bottom panels inaanddshow the coincident counts measured in the linear, the diagonal and the circular basis angles, respectively: H, horizontal; V, vertical; D, diagonal; D′ orthodiagonal; R, right; L, left. The averaged accumulation times for the histograms measured at E=18 and 29.2 kV cm−1were 160 and 200 min, respectively. Figure 4d depicts the results of the polarization-resolved photon correlation measurements when the electric field decreased to 18 kV cm −1 , where the corresponding Δ FSS was 30 μeV. Under these conditions, there is a high probability of generating a pair of photons with the same linear polarization, as shown in Figure 4e . No significant polarization correlation was observed in the diagonal and the circular bases. Hence, the fidelity under these conditions is below 0.5 ( Fig. 4f ), which shows that the two-photon state at 18 kV cm −1 is classically polarization correlated. Figure 4: Second-order cross-photon correlation histograms of biexciton–exciton photons. ( a ) Exciton and biexciton coincident counts for E=29.2 kV cm −1 (Δ FSS ~0) as a function of the delay time. The black dotted lines represent the coincident counts measured for photons of the same polarization, and the solid red lines show the orthogonal polarizations. ( b ) Degree of correlation C at E=29.2 kV cm −1 for the linear (top), the diagonal (middle) and the circular (bottom) bases. ( c ) Fidelity f + for several central pulse periods at E=29.2 kV cm −1 . ( d ) Exciton and biexciton coincident counts for E=18 kV cm −1 (Δ FSS =30 μeV) as a function of the delay time. The black dotted lines represent the coincident counts measured for photons of the same polarization, and the solid grey lines show the orthogonal polarizations. ( e ) Degree of correlation C at E=18 kV cm −1 for the linear (top), the diagonal (middle) and the circular (bottom) bases. ( f ) Fidelity f + for several central pulse periods at E=18 kV cm −1 . The QD was excited quasi-resonantly by the 740 nm laser energy to minimize the recapture of the carriers into the dot. The black dotted histograms in a and d are time-shifted for clarity. The top, the middle and the bottom panels in a and d show the coincident counts measured in the linear, the diagonal and the circular basis angles, respectively: H, horizontal; V, vertical; D, diagonal; D′ orthodiagonal; R, right; L, left. The averaged accumulation times for the histograms measured at E=18 and 29.2 kV cm −1 were 160 and 200 min, respectively. Full size image The above results demonstrate that the two-photon state emitted from the same GaAs QD can be manipulated from the polarization-correlated state to a polarization-entangled state by applying a vertical electric field. Because these GaAs island QDs emit light at a short wavelength (~750 nm), they will be useful for efficient detection of photons with silicon detectors. The reduction in Δ FSS for these dots, caused by the forward bias voltage, may also allow the fabrication of an efficient visible light-emitting diode, which can emit entangled photons with a high emission probability that is suitable for qubit-based optical [30] and spin [31] quantum computation applications. Quantum dots and device fabrication The sample consists of a 14-monolayer GaAs QW sandwiched between 25-nm-thick Al 0.3 Ga 0.7 As barriers and covered with a 50-nm-thick GaAs cap layer. A 2-min growth interruption was performed on both sides of the GaAs QW. This QW structure was grown on top of a 100-nm-thick undoped GaAs layer deposited on a 300-nm-thick n-GaAs layer ( n =1.5×10 17 cm −3 ). All layers were epitaxially grown by molecular beam epitaxy on an n-GaAs (100) substrate, which was used as a backside electrode. A Ti/Au film with an aperture of 200 nm in diameter was deposited on the sample surface to form a Schottky contact. The electric field is defined as E=( V g − V 0 )/ d , where V g is the applied gate voltage, V 0 is the Schottky barrier height (=0.93 V) obtained from independent photocurrent measurements, and d is the distance between the sample surface and the bottom n-doped GaAs layer ( d =205 nm). Optical spectroscopy measurements We focused the laser and collected the luminescence using a microscope objective lens with a numerical aperture of 0.4. A continuous wave and pulsed (6 ps) Ti:Al 2 O 3 laser was used for the excitation. The PL spectra were analysed by using a 55-cm-long monochromator coupled to an N 2 -cooled silicon charge-coupled device detector. A spectral notch filter was used to suppress the laser emission. Most of the QDs across the sample had line widths of ~120 μeV and were limited mainly by our set-up resolution. In the photon correlation measurements, the Hanbury Brown and Twiss (HBT) set-up was used to generate the photon correlation histograms with various polarization combinations. The collected PL was divided into two orthogonal detection arms using a 50/50 nonpolarizing pellicle beam splitter. Each arm of the HBT set-up was equipped with a single monochromator to filter the PL emission individually, in addition to a high-sensitivity avalanche photodiode. The electrical pulses from the two avalanche photodiodes were used to start and to stop a time-to-amplitude converter. The data within ±2.5 ns of were integrated to extract the total number of counts. For all optical measurements, the sample temperature was T =4 K. A combination set of half-wave and quarter-wave plates was inserted in the collection path of the HBT set-up for proper polarization state selection. No background subtraction or filtering was performed. The fidelity f + to the Bell state was calculated by measuring the correlation function for each polarization basis of the linear, diagonal and circular types [29] , where and are the second-order correlation functions when a biexciton photon is detected with a co-polarized and a cross-polarized exciton photon, respectively. The f + is expressed as: where C linear , C diagonal and C circular are the degrees of polarization correlation between the two emitted photons in the linear, the diagonal and the circular bases, respectively. How to cite this article: Ghali, M. et al . Generation and control of polarization-entangled photons from GaAs Island quantum dots by an electric field. Nat. Commun. 3:661 doi: 10.1038/ncomms1657 (2012).